Dynamical spin–orbital correlation in the frustrated magnet Ba3CuSb2O9 At low temperatures, atomic magnetic moments usually exhibit some order, for example ferromagnetic order. An exception is frustrated magnets, in which the symmetry impedes the minimization of energy by pairwise magnetic interactions. In such frustrated magnets, new quantum phases, such as spin liquids, are expected. Theoretically, a quantum liquid based on the orbital degree of freedom has also been considered possible when spin and orbital degrees of freedom are entangled. However, to date, experimental observation of such a dynamic spin–orbital state has been a challenge. Here we report an X-ray scattering study of a dynamic spin–orbital state in the frustrated magnet Ba 3 CuSb 2 O 9 . Orbital dynamical motion and increasing short-range orbital correlation with cooling are observed. The most significant feature is that the temperature variation of the orbital correlation is clearly affected by the magnetic interaction. This finding strongly supports a new quantum state in which spins and orbitals are entangled. Frustrated magnets have been widely studied, and various novel quantum phases have been predicted [1] , [2] , [3] . In a similar fashion, orbital degrees of freedom are often frustrated because of the strong anisotropy of the orbital coupling [4] , [5] , [6] , [7] . The orbital degree of freedom is relevant when electron orbitals with the same energy are occupied, and is often seen in transition metal oxides. For example, a Cu 2+ ion has nine 3 d electrons, and there is a degree of freedom in which one of the 3 d orbitals is left unoccupied. The coupling between the two frustrated degrees of freedom may lead to exotic states of matter. Motivated by such expectations, spin–orbital quantum liquid states have been extensively discussed for materials such as the triangular lattice magnet LiNiO 2 (refs 8 , 9 , 10 , 11 ) and the spinel FeSc 2 S 4 (ref. 12 ). However, in these compounds, spin and/or orbitals are found frozen at low temperatures [13] , [14] , [15] . The spin and orbital are usually decoupled because the orbital interaction is typically one order of magnitude stronger than the magnetic. If frustrated spins and degenerate orbitals have similar energy scales, the interaction between them may lead to a new quantum phase. A recent report [16] on a spin–orbital short-range order in the honeycomb-based magnet Ba 3 CuSb 2 O 9 provides a chance to study such a novel quantum state. The crystal structure of Ba 3 CuSb 2 O 9 is shown in Fig. 1 . The Cu and Sb are disordered in the yellow octahedra, and they form a short-range (~1 nm) honeycomb-based lattice [16] . Magnetic susceptibility shows that the magnetic interaction, J , is around 50 K. While some spins form spin singlets at around 50 K, the system exhibits gapless spin-liquid behaviour without forming any symmetry-breaking state down to 0.02 K (ref. 16 ). Therefore, the magnetism in this compound is highly frustrated. The orbital interaction energy is expected to be small because of the indirect connection of CuO 6 octahedra and the Cu-Sb dumbbell structure [16] . As a result, a long-range ferro-orbital ordering, which induces the symmetry change from hexagonal to orthorhombic, has been reported in slightly off-stoichiometric Ba 3 Cu 1− δ Sb 2+ δ O 9 at temperatures as low as 200 K (ref. 16 ). This temperature sets the characteristic scale for the orbital energy in this compound, and is not far from the magnetic energy scale, zJ ~180 K, where z is the coordination number [16] . Therefore, we expect a noticeable degree of interaction between the orbital and spin systems, resulting in a new quantum phase that involves both spins and orbitals. 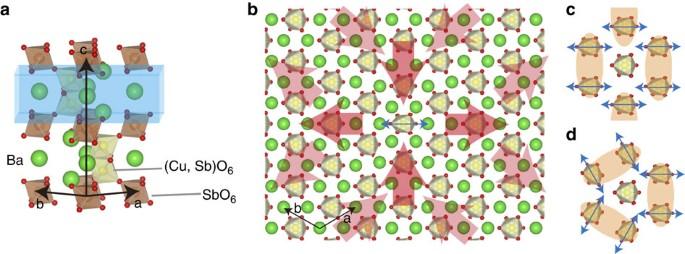Figure 1: Structure of Ba3CuSb2O9. (a) Crystal structure of Ba3CuSb2O9. (b) Strain field induced by a JT-distorted CuO6octahedron within thec-plane boxed ina. (c) Ferro-orbital cluster and (d) honeycomb orbital order cluster. Blue arrows show the direction of the octahedron distortion, and orange ellipses denote possible singlet pairs in a larger cluster. Figure 1: Structure of Ba 3 CuSb 2 O 9 . ( a ) Crystal structure of Ba 3 CuSb 2 O 9 . ( b ) Strain field induced by a JT-distorted CuO 6 octahedron within the c -plane boxed in a . ( c ) Ferro-orbital cluster and ( d ) honeycomb orbital order cluster. Blue arrows show the direction of the octahedron distortion, and orange ellipses denote possible singlet pairs in a larger cluster. Full size image In this paper, we experimentally investigate the spatial and temporal correlation of the orbital degree of freedom in hexagonal Ba 3 CuSb 2 O 9 using the long-range strain field caused by the Jahn-Teller (JT) distortion as an indicator of orbital occupancy. In the hexagonal phase, the average structure of CuO 6 octahedra has three-fold symmetry. However, the local structure violates this symmetry, as extended X-ray absorption fine structure (EXAFS) measurements have found temperature-independent JT distortion of the octahedra [16] . Every single CuO 6 octahedron with a static JT distortion makes a strain field as shown in Fig. 1b , which can be treated as a strain field around a point defect. Such a strain field gives rise to diffuse, Huang, scattering around the Bragg peaks with a significant anisotropy that reflects the symmetry of the strain field [17] , [18] , [19] . Here we report the observation of dynamical spin–orbital correlation in this compound through analysis of the Huang scattering. We found a clear saturation of the orbital correlation at the formation temperature of spin-singlet dimers, which strongly suggests entanglement between the spin and orbital degrees of freedom. Both the dynamic orbital correlation and temperature dependence of the local orbital arrangement indicate formation of a spin–orbital resonant state [16] , [20] . 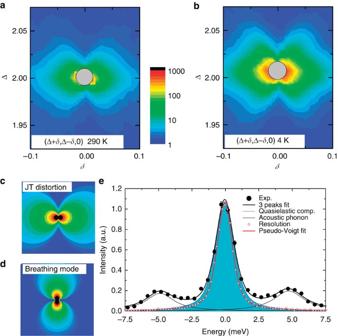Figure 2: Diffuse scattering aroundhh0 Bragg reflection. Intensity distribution around the 220 Bragg reflection measured at (a) 290 K and (b) 4 K. Calculated Huang diffuse intensity induced (c) by a JT mode distortion and (d) by a breathing mode distortion. Elastic constants for the calculation were obtained from inelastic X-ray scattering results (see Methods). All the maps present the intensity in a log scale. (e) Inelastic X-ray scattering spectrum of the diffuse intensity measured (4.2 3.8 0) at room temperature. Turquoise colouring highlights the quasielastic scattering component. a.u., arbitrary unit. The error bars are defined as the square root of the counted photon number, that is, the statistical error of the photon counting. Diffuse scattering from dynamical distortion Figure 2a shows the observed intensity distribution around the 220 Bragg reflection at 290 K. This reflection remains un-split down to 4 K, demonstrating the hexagonal symmetry of this crystal. We clearly see anisotropic diffuse intensity with lobes along the (horizontal) direction. The overall intensity distribution coincides with what is expected for Huang scattering caused by the JT distortion ( Fig. 2c ), and differs from the intensity distribution caused by the breathing mode distortion due to the difference in ionic sizes of Cu 2+ and Sb 5+ ( Fig. 2d ). This shows that the JT-distorted CuO 6 octahedra, or the anisotropic Cu 3 d orbitals, create a strong lattice strain field characterized by the mode shown in Fig. 1b. The intensity of the Huang scattering is so strong that the thermal diffuse scattering, which is induced by phonons and has less anisotropy 21 , is overwhelmed. Figure 2: Diffuse scattering around hh 0 Bragg reflection. Intensity distribution around the 220 Bragg reflection measured at ( a ) 290 K and ( b ) 4 K. Calculated Huang diffuse intensity induced ( c ) by a JT mode distortion and ( d ) by a breathing mode distortion. Elastic constants for the calculation were obtained from inelastic X-ray scattering results (see Methods). All the maps present the intensity in a log scale. ( e ) Inelastic X-ray scattering spectrum of the diffuse intensity measured (4.2 3.8 0) at room temperature. Turquoise colouring highlights the quasielastic scattering component. a.u., arbitrary unit. The error bars are defined as the square root of the counted photon number, that is, the statistical error of the photon counting. Full size image To clarify whether the orbital fluctuation is dynamic or static, we performed an inelastic X-ray scattering measurement at room temperature in the quasielastic scattering region [22] . Figure 2e presents the spectrum measured at (4.2 3.8 0), which is on the lobe of the Huang scattering around the 440 reflection, together with the instrumental resolution profile. The signals at ±5 meV are caused by the acoustic phonons, and the central quasielastic component is the Huang scattering. While random chemical disorder produces a monotonic elastic background, such a signal is at least one order of magnitude weaker than the quasielastic signal observed in this figure. A 3-peak fitting (pseudo-Voigt function for the central peak and Lorentzians for acoustic phonon peaks) performed on the spectrum yields 1.67(5) meV for the full width at half maximum of the quasielastic component, while the instrumental resolution is 1.36(5) meV. The intrinsic peak width of the diffuse intensity is 0.35(10) meV, which corresponds to a 2-ps lifetime for the orbital motion, and is, therefore, slower than the typical oxygen vibration frequency of a JT-distorted octahedron. This may be the result of spin–orbital coupling, as we will discuss. Temperature variation of orbital correlation The diffuse intensity shows noticeable temperature variation. Figure 2b shows the diffuse intensity measured at 4 K. It is stronger than that at 290 K for every region measured. This result means that the magnitude of the strain field increases with cooling, whereas the degree of JT distortion in each octahedron is temperature-independent [16] . The diffuse scattering intensity reflects the Fourier transform of the strain field. Assuming that the whole strain field is represented by the sum of the lattice distortion due to each orbital in the crystal, the diffuse intensity at the scattering vector Q is written as where ρ α ( r m ) denotes the occupancy of orbital α of the m -th site at position r m , t α ( q ) denotes the Fourier transform of the strain induced by the orbital α at the origin with q the deviation of Q from the reciprocal point nearby, and N denotes the number of orbitals in the sample. The sum over m is taken over the whole crystal, and provides the Fourier transform of the pair correlation function of the orbitals ‹ ρ α ( 0 ) ρ β ( r )›. The asterisk denotes the complex conjugate. A static isolated point defect at the origin creates a strain field proportional to | r | − 2 for large values of | r | (ref. 17 ). As a result, the radial dependence of | t ( q )| and the amplitude from a single orbital, F ( Q )= Q ˙ t α ( q ), are proportional to q −1 for small values of q =| q | while their angular dependence is governed by the symmetry of the orbital, as well as the elastic constants. For a random orbital distribution, the real space pair correlation function ‹ ρ α ( 0 ) ρ β ( r )› is δ r , 0 δ α , β , which means that the Q -space orbital pair correlation function is constant. This makes the intensity proportional to | F ( Q )| 2 , as shown in Fig. 2c. As the radial dependence of | F ( Q )| 2 is proportional to 1/ q 2 , the pair correlation function along a line through the Γ point is found by plotting the intensity multiplied by q 2 . Such a plot eliminates not only the uncorrelated part but also the thermal diffuse scattering, because it also has a 1/ q 2 dependence in the small q region. In Fig. 3a , we plot the experimentally observed intensity multiplied by q 2 for 290 and 4 K, together with that calculated for non-correlated orbitals (c). For a random orbital distribution, the contour plot shows no radial dependence, and only the angular distribution remains as shown in Fig. 3c . By contrast, both panels Fig. 3a show a peak centred at q =0, corresponding to a finite orbital correlation. 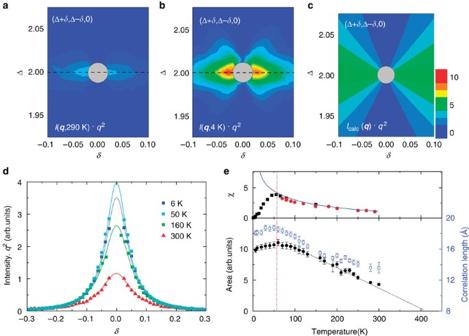Figure 3: Orbital correlation extracted fromI . q2. Contour map of (a)I(q,290K)q2and (b)I(q,4K)q2within thehk0-plane centred at the 220 Bragg point on a linear scale. (c) Contour map of the calculated intensity for non-correlated orbitals. (d) Line profiles along the dashed lines inaandbfor 6 K, 160 K and 300 K data after subtracting the background. Solid curves show the result of the Lorentzian fitting. (e) Temperature variation of the peak area (closed symbols) and the correlation length (open symbols) shown ind, together with the macroscopic magnetic susceptibility (solid line) and Knight shifts measured at magnetic fields of 12 T and 6 T reported in Quilliamet al.23in units of memu mol−1Oe−1(black squares and red circles). The dashed line at 55 K shows the similarity of the characteristic temperature of magnetism and that of orbital. arb. unit, arbitrary unit. The error bars show the standard errors of the parameters derived by the least squares fitting. Figure 3d shows the profiles along the dashed lines in Fig. 3a . It is clear that the correlation grows with decreasing temperature, and the correlation length, that is, the inverse peak width, increases up to 19 Å with cooling. Theoretically, finite orbital coupling is expected [20] through the antiferromagnetic coupling J . In this case, the typical energy scale of the magnetism-originated orbital motion is zJ ~180 K (ref. 16 ). As shown in Fig. 3e , the orbital correlation starts growing at ~400 K. The discrepancy between 180 and 400 K is attributable to the fluctuation of z , as z can vary between 0 and 9 from site to site. The order grows as the temperature decreases down to 50 K. The top panel shows the magnetic susceptibility obtained by both the NMR measurement and dc-susceptibility [23] , which shows the singlet formation for some of the spins around 50 K. The orbital correlation, whose characteristic energy scale is 200 K, is clearly affected by the magnetism with J ~50 K. Figure 3: Orbital correlation extracted from I . q 2 . Contour map of ( a ) I ( q ,290 K ) q 2 and ( b ) I ( q ,4 K ) q 2 within the hk 0-plane centred at the 220 Bragg point on a linear scale. ( c ) Contour map of the calculated intensity for non-correlated orbitals. ( d ) Line profiles along the dashed lines in a and b for 6 K, 160 K and 300 K data after subtracting the background. Solid curves show the result of the Lorentzian fitting. ( e ) Temperature variation of the peak area (closed symbols) and the correlation length (open symbols) shown in d , together with the macroscopic magnetic susceptibility (solid line) and Knight shifts measured at magnetic fields of 12 T and 6 T reported in Quilliam et al. [23] in units of memu mol −1 Oe −1 (black squares and red circles). The dashed line at 55 K shows the similarity of the characteristic temperature of magnetism and that of orbital. arb. unit, arbitrary unit. The error bars show the standard errors of the parameters derived by the least squares fitting. Full size image Based on this observation, we expect that the dynamical movement of the orbital observed at room temperature persists even at low temperature, and a quantum state that involves both spin and orbital occurs below 50 K in this compound. To test this idea, we used the diffuse intensity distribution to examine the structure of the orbital short-range order. The peak at the Γ-point in the I . q 2 map is caused by the ferro-orbital correlation shown in Fig. 1c , the same mode as the static JT distortion in the off-stoichiometric sample. In addition, excess intensity that emerged in cooling was observed in Fig. 2b around (Δ, δ )=(2±0.05,±0.05). The ferro-orbital correlation cannot reproduce such anisotropy in diffuse intensity, but the honeycomb orbital correlation in Fig. 1d and its inversion variant, which were proposed in Nakatsuji et al. [16] and Nasu et al. [20] , reproduce the feature as shown in Fig. 4a . The growth of the anisotropy in the intensity distribution, as well as the intensity around the Γ-point indicates increasing competition between the antiferro- and ferro-orbital orders with decreasing temperature. 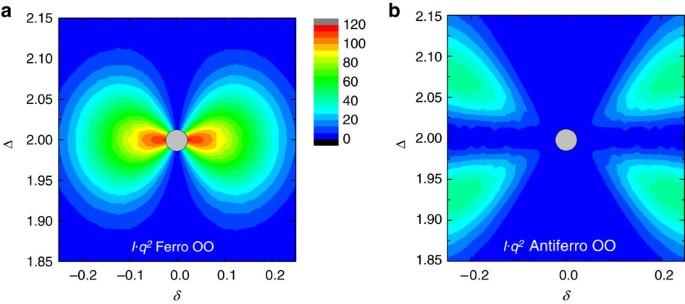Figure 4: Calculated diffuse intensity multiplied byq2for ferro- and antiferro-orbital order clusters. Contour map of calculatedI(q) .q2around 220 Bragg reflection for (a) ferro-orbital clusters shown inFig. 1cand (b) honeycomb orbital clusters shown inFig. 1d. Figure 4: Calculated diffuse intensity multiplied by q 2 for ferro- and antiferro-orbital order clusters. Contour map of calculated I ( q ) . q 2 around 220 Bragg reflection for ( a ) ferro-orbital clusters shown in Fig. 1c and ( b ) honeycomb orbital clusters shown in Fig. 1d . Full size image Our results show that the orbitals fluctuate with correlation down to much lower temperature than the orbital energy scale. Figure 1c show the experimentally observed orbital structures, in which two adjacent orbitals align ferroically to form a spin-singlet pair. This arrangement supports recent theoretical work on this compound [20] , [24] that predicts an entanglement between spins and orbitals. From a calculation for a small cluster [20] , the theory derives the resonant state of the orbital arrangement shown in Fig. 1d and its inversion variant with a typical time scale of 1–10 ps. All of these agree with our measurements. The experimentally observed ferro-orbital correlation may be caused by the large system size of the real crystal, which is not taken into account in the theory. When the entangled state is established, the growth of the orbital correlation is expected to saturate, just as we observe ( Fig. 3e ). Another interpretation of the saturation would be orbital freezing or an orbital glass transition. However, there is no corresponding signal in the specific heat [25] , [16] or NMR (ref. 23 ) around 50 K. In summary, we performed a series of X-ray scattering experiments on the frustrated system Ba 3 CuSb 2 O 9 , and found competing ferro- and antiferro-orbital fluctuations. The two fluctuations develop with cooling, and the ferro-orbital correlation saturates at the spin-singlet formation temperature. This saturation implies the formation of a spin–orbital entangled state in the hexagonal Ba 3 CuSb 2 O 9 . We note that the method used here to study the orbital correlation is based on the observation of the strain field induced by the JT effect, thus is applicable to other orbitally fluctuating JT systems. In particular, e g electron systems of octahedral coordinated compounds, such as Mn 3+ and Cu 2+ oxides, would provide strong signal intensity because of their large orbital-lattice coupling. Sample Single crystals of Ba 3 CuSb 2 O 9 were grown by the flux method. The sample studied in this study keeps hexagonal symmetry down to 4 K. Diffuse X-ray scattering The diffuse X-ray scattering measurements on the obtained crystal with dimensions of 0.4 × 0.3 × 0.05 mm were performed with 12 keV X-rays using four-circle diffractometers at BL-3A and BL-4C of the Photon Factory, KEK, Japan. The temperature dependence measurements were performed with a closed cycle refrigerator in a warming process. Inelastic X-ray scattering The inelastic X-ray scattering measurements with 21.747 keV X-rays were conducted at BL35XU of SPring-8 in Japan [26] . The energy resolution was determined using scattering from polymethyl methacrylate. Pseudo-Voigt fitting gave the full width at half maximum of 1.36(5) meV as shown in Fig. 2e . Calculation of diffuse scattering The calculation of the diffuse intensity was done with elastic constants c 11 =320 GPa and c 12 =209 GPa, which were obtained from the inelastic X-ray scattering measurements. Equal amounts of three orbital domains that are connected by 120° rotation about the c -axis were assumed. How to cite this article: Ishiguro, Y. et al. Dynamical spin–orbital correlation in the frustrated magnet Ba 3 CuSb 2 O 9 . Nat. Commun. 4:2022 doi: 10.1038/ncomms3022 (2013).